Sequence-regulated vinyl copolymers by metal-catalysed step-growth radical polymerization Proteins and nucleic acids are sequence-regulated macromolecules with various properties originating from their perfectly sequenced primary structures. However, the sequence regulation of synthetic polymers, particularly vinyl polymers, has not been achieved and is one of the ultimate goals in polymer chemistry. In this study, we report a strategy to obtain sequence-regulated vinyl copolymers consisting of styrene, acrylate and vinyl chloride units using metal-catalysed step-growth radical polyaddition of designed monomers prepared from common vinyl monomer building blocks. Unprecedented ABCC-sequence-regulated copolymers with perfect vinyl chloride–styrene–acrylate–acrylate sequences were obtained by copper-catalysed step-growth radical polymerization of designed monomers possessing unconjugated C=C and reactive C–Cl bonds. This strategy may open a new route in the study of sequence-regulated synthetic polymers. One of the ultimate goals of synthetic polymer chemistry is to obtain sequence-regulated polymers, which are often observed in natural macromolecules such as proteins and nucleic acids. For this purpose, various synthetic approaches have been developed, such as Merrifield's solid-phase synthesis and enzymatic or non-enzymatic template polymerization, which are used for the synthesis of oligopeptides and oligonucleotides from natural or non-natural building blocks and for producing non-natural oligoamides, oligoesters, oligoureas, oligocarbamates and oligosaccharides [1] , [2] , [3] , [4] , [5] , [6] , [7] , [8] , [9] , [10] . These are all condensation polymers consisting of heteroatom-containing main-chain linkages, such as amide, ester, ether and so on, and prepared by successive stepwise condensation reactions, which can be automated sometimes [2] , [3] . In contrast, sequence control in vinyl polymerization, which produces stable C–C bond-linked polymers, is much more difficult because the polymerization proceeds through a chain-growth mechanism in which the step-by-step addition of monomers with a controlled sequence is basically impossible. In radical copolymerization, propagation statistically occurs according to monomer reactivity ratios to generally result in statistical or random copolymers ( Fig. 1a ) [11] . Although some monomer pairs with favourable cross-propagation parameters predominantly produce alternating copolymers to enable a kind of sequence regulation, the sequence control is limited to the AB sequence and is not perfect. A combination of living polymerization and the sequential monomer addition technique has been used for sequence-regulated vinyl oligomers and polymers [12] , [13] , [14] , whereas the perfect sequence regulation has not been attained because of the inevitable chain reaction of added monomers. Meanwhile, there are several methodologies to obtain the equivalents of sequence-regulated vinyl copolymers. Polymerizations of substituted dienes or their copolymerization and ring-opening metathesis polymerizations or acyclic diene polymerizations, followed by hydrogenation, were used for the synthesis of linear copolymers of ethylene and polar vinyl monomers, in which the functional groups are periodically located in the main chain, although regio-irregularity is inevitable because of mechanisms such as 1,2- or 3,4-insertion for diene polymerization and equivalents of head-to-head sequence for metathesis polymerizations [15] , [16] , [17] , [18] . 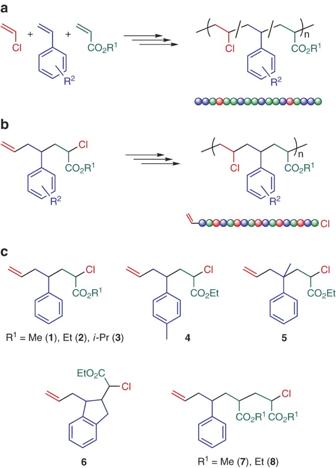Figure 1: The concept of metal-catalysed step-growth radical polymerization of designed monomers for sequence-regulated vinyl copolymers. (a) Chain-growth radical copolymerization of vinyl monomers results in random or statistical copolymers depending on the monomer reactivity ratio. (b) Step-growth radical polymerization of designed monomers with unconjugated C=C and reactive C–Cl bonds to yield ABC-sequence-regulated copolymers. (c) Designed abc- (1–6) and abcc monomers (7and8) prepared from common vinyl monomers as building blocks for completely sequence-regulated vinyl copolymers with styrenes, acrylates and vinyl chloride units. Figure 1: The concept of metal-catalysed step-growth radical polymerization of designed monomers for sequence-regulated vinyl copolymers. ( a ) Chain-growth radical copolymerization of vinyl monomers results in random or statistical copolymers depending on the monomer reactivity ratio. ( b ) Step-growth radical polymerization of designed monomers with unconjugated C=C and reactive C–Cl bonds to yield ABC-sequence-regulated copolymers. ( c ) Designed abc- ( 1 – 6 ) and abcc monomers ( 7 and 8 ) prepared from common vinyl monomers as building blocks for completely sequence-regulated vinyl copolymers with styrenes, acrylates and vinyl chloride units. Full size image This article describes a new approach to sequence-regulated vinyl copolymers through metal-catalysed step-growth radical polymerization of designed monomers ( Fig. 1b ) that are prepared from common vinyl monomer building blocks ( Fig. 1c ). We have recently developed the metal-catalysed radical polyaddition by evolution of metal-catalysed atom-transfer radical addition (ATRA) or Kharasch addition [19] into the step-growth polymerization of a designed monomer possessing an unconjugated C=C double bond and a reactive C–Cl bond [20] , [21] . This polymerization proceeds through a C–C bond forming reactions between the radical species generated through the metal-catalysed activation of the C–Cl bond and the unconjugated C=C bond of another molecule to lead to linear polymers by step-growth propagation. We have succeeded in the synthesis of linear polyesters by step-growth radical polymerization of the designed monomers, the C=C and C–Cl bonds of which are linked by an ester linkage [21] . The polymerization addition reaction gives a –CH 2 –CHCl– motif, in which the C–Cl bond is unreactive towards the metal catalyst, in contrast to the original C–Cl bond of the monomer, which is adjacent to the carbonyl group. The newly formed –CH 2 –CHCl– unit is equivalent to the poly(vinyl chloride) repeating unit; this inspired us to construct sequence-regulated vinyl copolymers using step-growth radical polymerization of further designed monomers. We thus designed a series of new monomers consisting of unconjugated C=C and reactive C–Cl end groups, which are linked through C–C chains and prepared from commercially available common vinyl monomers (that is, styrenes and acrylates) through simple synthetic routes. This novel strategy based on the C–C bond-forming step-growth polymerization of prelinked monomers led to the formation of abc- and abcc-sequence-regulated vinyl monomers. abc Monomers We initially prepared a series of abc-type monomers ( Fig. 2a ) that may result in the completely sequence-regulated copolymers of vinyl chloride, styrenes and acrylates by step-growth radical polymerization. As for the sequence-regulated copolymers with a styrene and methyl acrylate unit, we first conducted RuCl 2 (PPh 3 ) 3 -catalysed ATRA between methyl dichloroacetate and styrene to almost quantitatively prepare the 1:1 adduct [22] . One of the C–Cl bonds, adjacent to the phenyl group, was subsequently and selectively activated by TiCl 4 to form the carbocation adjacent to the phenyl group, to which the vinyl group was introduced by allylation with allyltrimethylsilane in high yield [23] . A series of abc monomers with different ester substituents [methyl ( 1 ), ethyl ( 2 ) and isopropyl ( 3 )] and styrene derivatives [styrene ( 1 – 3 ), p -methylstyrene ( 4 ), α-methylstyrene ( 5 ) and indene ( 6 )] were obtained by the two-step simple reactions, followed by distillation, and characterized by 1 H, 13 C, H-H and H-C COSY NMR, MALDI-TOF-MS and ESI-MS, and elemental analysis ( Supplementary Figs. S1–S4 ), although the obtained monomers were mixtures of diastereomers with two asymmetric carbons. 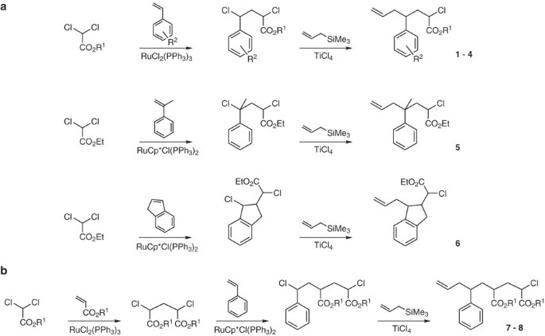Figure 2: Synthesis of designed monomers for sequence-regulated vinyl copolymers. (a) abc-Monomers (1–6) were prepared by ruthenium-catalysed Kharasch addition between alkyl dichloroacetate and styrene derivatives, followed by TiCl4-catalysed allylation of the C–Cl bond adjacent to the styrene unit with allyltrimethylsilane. (b) abcc-Monomers were prepared by double ruthenium-catalysed Kharasch addition between alkyl dichloroacetate with acrylate first and then with styrene, followed by TiCl4-catalysed allylation of the C–Cl bond adjacent to the styrene unit with allyltrimethylsilane. Figure 2: Synthesis of designed monomers for sequence-regulated vinyl copolymers. ( a ) abc-Monomers ( 1 – 6 ) were prepared by ruthenium-catalysed Kharasch addition between alkyl dichloroacetate and styrene derivatives, followed by TiCl 4 -catalysed allylation of the C–Cl bond adjacent to the styrene unit with allyltrimethylsilane. ( b ) abcc-Monomers were prepared by double ruthenium-catalysed Kharasch addition between alkyl dichloroacetate with acrylate first and then with styrene, followed by TiCl 4 -catalysed allylation of the C–Cl bond adjacent to the styrene unit with allyltrimethylsilane. Full size image Various metal (ruthenium, iron, copper) complexes effective for ATRA [19] and metal-catalysed living radical polymerization or atom-transfer radical polymerization [24] , [25] , [26] , [27] , [28] were then used for the step-growth radical polymerization of these abc monomers. The vinyl group and the C–Cl bond of the monomers were consumed with all the metal catalysts, although the rates and molecular weights of the products were dependent on both catalysts and monomers ( Supplementary Figs. S5–S7 ). Copper-based catalysts generally yielded higher molecular-weight products than ruthenium- and iron-based ones. On increasing the bulkiness of the ester substituent of monomers, the molecular weights of the products increased. A detailed analysis of the products revealed that they consisted of oligomers as major products synthesized through intermolecular polyaddition, and cyclic by-products through intramolecular cyclization of monomers ( Supplementary Fig. S8 ) [29] . The contents of cyclic compounds were estimated by size-exclusion chromatography (SEC) of the products by ultraviolet detection and the 1 H NMR spectra of the fractionated compounds around the monomer molecular-weight region. As summarized in Table 1 , the contents of the cyclic by-products remarkably decreased from 31 to 6% on increasing the bulkiness of the ester substituents from Me to i Pr. This indicates that a bulkier ester substituent suppresses the intramolecular cyclization of monomers to preferentially induce intermolecular polyaddition, resulting in higher molecular-weight products. In contrast, rigid α-methylstyrene or indene units slightly increased the cyclic compound. Thus, the design of monomers is important for an efficient step-growth polymerization, leading to sequence-regulated polymers with higher molecular weights. Table 1 Metal-catalysed step-growth radical polymerization of abc and abcc monomers. Full size table abcc Monomers To reduce the intramolecular cyclization of monomers, we built abcc-type monomers ( 7 ) by adding one more vinyl monomer unit to the abc monomers so that the C=C and C–Cl units can be distantly located. The molecular models optimized by MOPAC also suggest that this strategy might be appropriate for this purpose ( Supplementary Fig. S9 ). The abcc-type monomer consisting of one styrene and two methyl acrylate units was synthesized by the sequential ruthenium-catalysed ATRA of methyl acrylate and styrene, both of which are common vinyl monomers, in this order to methyl dichloroacetate, followed by allylation to the styrene unit ( Fig. 2b ). The products were isolated by distillation and characterized by 1 H, 13 C ( Fig. 3a ), H-H and H-C COSY NMR, MALDI-TOF-MS and ESI-MS, and elemental analysis ( Supplementary Figs. S10–S12 ). 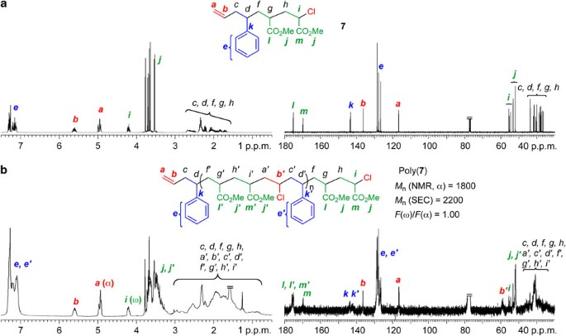Figure 3:1H and13C NMR spectra of the abcc-monomer and the ABCC-sequence-regulated copolymer. (a)1H and13C NMR spectra of7. (b)1H and13C NMR spectra of poly(7) obtained with CuCl/N,N,N′,N″,N″-pentamethyldiethylenetriamine (PMDETA) ([CuCl]0=200 mM; [PMDETA]0=800 mM) in bulk at 100 °C. All spectra were measured in CDCl3at room temperature The brackets for repeating units in poly(7) are positioned differently from those inFigs. 1and4so that the signals originating from the terminal groups can be assigned to the chemical structures. Figure 3: 1 H and 13 C NMR spectra of the abcc-monomer and the ABCC-sequence-regulated copolymer. ( a ) 1 H and 13 C NMR spectra of 7 . ( b ) 1 H and 13 C NMR spectra of poly( 7 ) obtained with CuCl/ N , N , N′ , N″ , N″ -pentamethyldiethylenetriamine (PMDETA) ([CuCl] 0 =200 m M ; [PMDETA] 0 =800 m M ) in bulk at 100 °C. All spectra were measured in CDCl 3 at room temperature The brackets for repeating units in poly( 7 ) are positioned differently from those in Figs. 1 and 4 so that the signals originating from the terminal groups can be assigned to the chemical structures. Full size image This abcc-type monomer was thus polymerized by the copper catalyst ( Fig. 4a ). Both C=C and C–Cl bonds were simultaneously consumed at nearly the same rate, indicating the 1:1 reaction between these groups ( Fig. 4b ). Furthermore, a faster monomer molecule consumption measured by SEC with a ultraviolet detector than the C=C and C–Cl consumptions measured by 1 H NMR suggests that abcc monomers were predominantly consumed by intermolecular reaction rather than by intramolecular cyclization. In addition to these kinetic data, the SEC curve of the products shifted to higher molecular weights along with the reaction, also indicating that the intermolecular polymerization preferentially proceeded ( Fig. 4c ). A further analysis of the products showed that the content of intramolecularly cyclized monomers was below 2% ( Table 1 ), which was remarkably improved in comparison with the abc-type counterparts. A similar result was also obtained using abcc monomers with ethyl ester substituents ( 8 ) ( Table 1 and Supplementary Fig. S13 ). 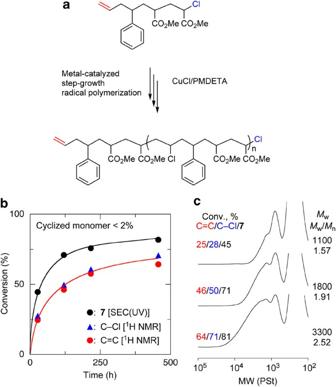Figure 4: Metal-catalysed step-growth radical polymerization of the abcc monomer. (a) Polymerization scheme of7with CuCl/N,N,N′,N″,N″-pentamethyldiethylenetriamine (PMDETA). (b) Conversion of monomer (7) measured by SEC with a ultraviolet detector and C–Cl and C=C bonds measured by1H NMR in metal-catalysed step-growth radical polymerization with CuCl/PMDETA in bulk at 60 °C; [7]0=bulk; [CuCl]0=200 mM; [PMDETA]0=800 mM. (c) SECs of the obtained polymers. Figure 4: Metal-catalysed step-growth radical polymerization of the abcc monomer. ( a ) Polymerization scheme of 7 with CuCl/ N , N , N′ , N″ , N″ -pentamethyldiethylenetriamine (PMDETA). ( b ) Conversion of monomer ( 7 ) measured by SEC with a ultraviolet detector and C–Cl and C=C bonds measured by 1 H NMR in metal-catalysed step-growth radical polymerization with CuCl/PMDETA in bulk at 60 °C; [ 7 ] 0 =bulk; [CuCl] 0 =200 m M ; [PMDETA] 0 =800 m M . ( c ) SECs of the obtained polymers. Full size image Formation of well-defined ABCC-sequence-regulated copolymers was also confirmed by the 1 H and 13 C NMR spectra of the products ( Fig. 3b ), which showed relatively broad peaks of the repeating units at almost the same chemical shifts as those of monomers ( Fig. 3a ). Furthermore, the terminal C=C and C–Cl bonds almost completely remained. The number-average molecular weights ( M n ) calculated from the peak intensity ratios of the end groups to the main-chain protons were exactly the same [ M n (C=C)= M n (C–Cl)=1,800] and similar to those obtained by SEC [ M n (SEC)=2,200], suggesting that most of the obtained oligomers and polymers did not cyclize and were linear. The formation of the structure equivalent to the vinyl chloride unit was also supported by 13 C NMR. Furthermore, the MALDI-TOF-MS spectrum showed a series of peaks separated by 339, equal to the mass of the abcc monomers ( Supplementary Fig. S14 ). These results indicated that the completely sequence-regulated ABCC-vinyl copolymers of the styrene–acrylate–acrylate–vinyl chloride units were obtained by metal-catalysed step-growth radical polymerization of abcc monomers, originally prepared from styrene and acrylate as building blocks. abc-Monomers were also polymerized by metal catalysts to yield ABC-sequence-regulated copolymers consisting of styrene–acrylate–vinyl chloride units, whereas the intramolecular cyclization of abc monomers could not be fully suppressed. Although the molecular weights are still relatively low as vinyl polymers, they may be high enough for some purpose, as observed with sequence-regulated functional oligoamides and oligopeptides. However, more effective catalysts should be developed in terms of activity and molecular weights. Another more challenging topic for this metal-catalysed radical polyaddition of the designed monomers would be precise molecular weight control, as in living polymerization. It is very difficult in principle because the reaction proceeds through a step-growth mechanism, in which addition reactions occur randomly among monomers, oligomers and polymers. However, it might be possible by monomer or catalyst design, which enables a selective activation of the C–Cl bond at oligomers or polymer chain ends rather than that in the monomer, in a similar way to chain-growth condensation polymerization [30] . In conclusion, this conceptually new synthetic approach based on step-growth C–C bond-forming polymerization leads to structures equivalent to various sequence-regulated vinyl copolymers consisting of stable C–C-bond main chains, which are completely different from sequence-regulated natural macromolecules, such as proteins and nucleic acids. The further design of monomers and catalysts can provide sequence-regulated C–C-linked polymers possessing functional groups with desired sequences, which could be used as novel functional synthetic macromolecules. Materials RuCp*Cl(PPh 3 ) 2 (Wako; 99%), FeCl 2 (Aldrich; 99.99%) and CuCl (Aldrich; 99.99%) were used as received and handled in a glove box (VAC Nexus) under a moisture- and oxygen-free argon atmosphere (oxygen <1 p.p.m.). Toluene was distilled over sodium benzophenone ketyl and bubbles with dry nitrogen for 15 min just before use. P n Bu 3 (KANTO, >98%) was used as received. N,N,N′,N″,N″ -Pentamethyldiethylenetriamine (TCI, >98%) and 1,1,4,7,10,10-hexamethyltriethylenetetramine (Aldrich, 97%) were distilled from calcium hydride before use. Monomer synthesis All monomers were prepared using Kharasch addition reactions initiated from various dichloroacetates, and common vinyl monomers as building blocks, with RuCl 2 (PPh 3 ) 3 or RuCp*Cl(PPh 3 ) 2 as catalysts, followed by allylation by allyltrimethylsilane with TiCl 4 . All reactions were carried out by the syringe technique under dry nitrogen in glass tubes equipped with a three-way stopcock. For typical examples, the procedures for preparing monomers 3 and 7 were described as follows: As the first step for the synthesis of 3 , dichloroacetyl chloride (300 ml, 3.11 mol) was added dropwise with vigorous stirring to a solution of 2-propanol (226 ml, 2.97 mol) and triethylamine (455 ml, 3.26 mol) in dry tetrahydrofuran (502 ml) at 0 °C. The mixture was stirred for 1 h at 0 °C and then over 24 h at room temperature. After dilution with diethyl ether, the mixture was washed with aqueous Na 2 CO 3 and then with NaCl solutions and was evaporated to remove the solvents. The product was distilled over calcium hydride under reduced pressure to yield pure isopropyl dichloroacetate (278 ml, 1.92 mol; yield=64.7%, purity >99%). In a 500 ml round-bottomed flask were placed RuCl 2 (PPh 3 ) 3 (2.08 g, 2.17 mmol), toluene (10.0 ml), styrene (50.0 ml, 0.434 mol) and isopropyl dichloroacetate (157 ml, 1.08 mol) at room temperature. The flask was placed in an oil bath maintained at 60 °C under vigorous stirring. The conversion of styrene was determined from the concentration of the residual styrene measured by gas chromatography, with toluene as an internal standard. After 40 h, the conversion of styrene reached 61% to form the 1:1 adduct almost quantitatively. After the precipitation of the ruthenium complex into n -hexane, the solvent was evaporated to yield the crude product. The 1:1 adduct was purified by distillation over CaH 2 (34.9 ml, 0.147 mol, 33.7%). To a dichloromethane solution of the adduct (34.9 ml, 0.147 mol) and allyltrimethylsilane (47.0 ml, 0.296 mol) was added 8.1 ml of TiCl 4 dropwise at −78 °C under dry nitrogen. The mixture was kept stirred for 4.5 h at −78 °C, and then over 80 h at 0 °C. The reaction was terminated with 2-propanol (20 ml) and the mixture was washed with aqueous HCl and NaOH solutions, and finally with water. The organic layer was evaporated to remove the solvents. Monomer 3 was purified by distillation over CaH 2 to yield a clear and colourless viscous oil (total yield 13.6%, purity >99%). C 16 H 21 ClO 2 (280.79): calcd. carbon 68.44, hydrogen 7.54, chlorine 12.63; found carbon 68.33, hydrogen 7.55, chlorine 12.60. As the first step for the synthesis of 7 , in a 500 ml round-bottomed flask were placed RuCl 2 (PPh 3 ) 3 (3.72 g, 3.88 mmol), toluene (18.0 ml), methyl acrylate (70.0 ml, 0.78 mol) and methyl dichloroacetate (300 ml, 2.90 mol) at room temperature. The flask was placed in an oil bath kept at 80 °C under vigorous stirring. The conversion of methyl acrylate was determined from the concentration of the residual methyl acrylate measured by gas chromatography, with toluene as an internal standard. After 90 h, the conversion of methyl acrylate reached 93% to form the 1:1 adduct almost quantitatively. After the precipitation of the ruthenium complex into hexane, the solvent was evaporated to yield the crude product. The 1:1 adduct was purified by distillation over CaH 2 (82.0 ml, 0.491 mol, 63.3%). The Kharasch addition reaction between styrene and the adduct was carried out similarly. In a 200 ml round-bottomed flask were placed RuCp*Cl(PPh 3 ) 2 (0.430 g, 0.540 mmol), toluene (4.0 ml), styrene (24.0 ml, 0.209 mol) and the adduct (80.0 ml, 0.478 mol) at room temperature. The flask was placed in an oil bath maintained at 60 °C under vigorous stirring. The conversion of styrene was determined from concentration of the residual styrene measured by 1 H NMR, with toluene as an internal standard. After 64 h, the conversion of styrene reached 85% to form the 1:1 adduct almost quantitatively. To remove the ruthenium complex, the reaction mixture was led to pass through a silica-gel column eluted with n -hexane and diethyl ether, and then evaporated in vacuum to yield the crude product (61.3 ml, 0.184 mol, 85.0%). To a dichloromethane solution of the adduct (80.0 ml, 0.312 mol) and allyltrimethylsilane (95 ml, 0.599 mol) was added 16.5 ml of TiCl 4 dropwise at −78 °C under dry nitrogen. The mixture was stirred for 2 h at −78 °C, and then over 40 h at 0 °C. The reaction was terminated with methanol (40 ml) and the mixture was washed with aqueous HCl and then with NaOH solutions, and finally with water. The organic layer was evaporated to remove the solvents. Monomer 7 was purified by distillation over CaH 2 to yield pure 7 as a clear and colourless viscous oil (total yield 24.6%, purity >99%). C 18 H 23 ClO 4 (338.83): calcd. carbon 63.81, hydrogen 6.84, chlorine 10.46; found carbon 63.36, hydrogen 6.82, chlorine 10.31. Polymerizations Polymerization was carried out under dry nitrogen in baked glass tubes equipped with a three-way stopcock. A typical example of the polymerization procedure is given below. To a suspension of CuCl (59.4 mg, 0.60 mmol) in toluene (2.20 ml) was added N , N , N′ , N″ , N″ -pentamethyldiethylenetriamine (0.48 ml, 2.40 mmol), and the mixture was stirred for 12 h at 80 °C to yield a heterogeneous solution of the CuCl/ N , N , N′ , N″ , N″ -pentamethyldiethylenetriamine complex. After the solution was cooled to room temperature, monomer ( 7 ) (5.50 ml, 0.195 mol) was added to yield homogeneous solutions. The solution was evenly charged in 12 glass tubes and the tubes were sealed by flame under nitrogen atmosphere. The tubes were immersed in a thermostatic oil bath at 60 °C. At predetermined intervals, the polymerization process was terminated by cooling the reaction mixtures to −78 °C. The conversions of the functional groups (C=C and C–Cl) of 7 were determined from the residual concentrations of C=C and C–Cl by 1 H NMR spectroscopy, with toluene as an internal standard. Measurements Monomer conversion was determined from the concentration of residual monomer by SEC equipped with a ultraviolet detector. The conversions of the functional groups (C=C and C–Cl) of monomers were determined from the concentration of C=C and C–Cl by 1 H NMR spectroscopy, with toluene as an internal standard. 1 H NMR spectra were recorded in CDCl 3 at 25 °C on a JEOL ECS–400 spectrometer, operating at 400 MHz. The M n and weight-average molecular weight ( M w ) of the product polymers were determined by SEC in tetrahydrofuran at 40 °C on two polystyrene gel columns (Shodex K-805L (pore size: 20–1,000 Å; 8.0 mm i.d. ×30 cm) ×2; flow rate 1.0 ml min −1 ) connected to a Jasco PU-980 precision pump and a Jasco 930-RI detector. The columns were calibrated against eight standard polystyrene samples (Shodex; M p =526–900,000; M w / M n =1.01–1.14). MALDI-TOF-MS spectra were measured on a Shimadzu AXIMA-CFR Plus mass spectrometer (linear mode) with dithranol (1,8,9-anthracenetriol) as the ionizing matrix and sodium trifluoroacetate as the ion source. ESI-MS spectra were recorded on a JEOL JMS-T100CS spectrometer. Molecular modelling and molecular mechanics (MM) calculations were implemented in the Scigress Workspace (version 7.6) operated using a PC running under Windows ® XP. The structures were optimized first with MM2 and then with AM1 in MOPAC. How to cite this article: Satoh, K. et al . Sequence-regulated vinyl copolymers by metal-catalysed step-growth radical polymerization. Nat. Commun. 1:6 doi: 10.1038/ncomms1004 (2010).